Monosynaptic inputs to new neurons in the dentate gyrus Adult hippocampal neurogenesis is considered important for cognition. The integration of newborn dentate gyrus granule cells into the existing network is regulated by afferent neuronal activity of unspecified origin. Here we combine rabies virus-mediated retrograde tracing with retroviral labelling of new granule cells (21, 30, 60, 90 days after injection) to selectively identify and quantify their monosynaptic inputs in vivo . Our results show that newborn granule cells receive afferents from intra-hippocampal cells (interneurons, mossy cells, area CA3 and transiently, mature granule cells) and septal cholinergic cells. Input from distal cortex (perirhinal (PRH) and lateral entorhinal cortex (LEC)) is sparse 21 days after injection and increases over time. Patch-clamp recordings support innervation by the LEC rather than from the medial entorhinal cortex. Mice with excitotoxic PRH/LEC lesions exhibit deficits in pattern separation but not in water maze learning. Thus, PRH/LEC input is an important functional component of new dentate gyrus neuron circuitry. Adult neurogenesis has become an increasingly well-accepted phenomenon in mammals including humans. Neurogenesis is deemed limited to two areas: the subventricular zone which gives rises to new olfactory neurons and the dentate gyrus(DG) [1] . New neurons derived from neural progenitor cells are added daily to the DG. A subset of these new neurons survives and gradually integrates into the hippocampal network [1] . During maturation, newborn granule cells (GCs) exhibit enhanced plasticity [2] , [3] , [4] . Continuous addition of easily excitable new neurons to the DG suggests a unique contribution of neurogenesis to memory function [5] . Indeed, studies ablating or enhancing adult neurogenesis followed by behavioural testing have revealed a role for newborn GCs in fine pattern separation attributed to the DG [6] , [7] , [8] . However, the neural circuits that regulate the function of newborn GCs remain unresolved. To identify the neuronal network that regulates the integration of newborn GCs and to understand the functional significance of adult neurogenesis, it is essential to define direct afferent inputs of new neurons. In particular, it is not known if the circuits into which new GCs are integrated to process information, differ from those of mature DG cells. To achieve this aim, we developed a dual-virus approach using a novel monosynaptic rabies virus-mediated retrograde tracing system [9] . First, retrovirus (RV-SYN-GTRgp) expressing nucleus-localized green fluorescent protein (GFP), TVA receptor and rabies glycoprotein (Rgp) under control of the synapsin promoter was injected into the DG to label only dividing neural progenitor cells, that differentiate into new GCs over time. Second, EnvA-pseudotyped rabies virus, in which Rgp was replaced with mCherry (EnvA-ΔG-MCh), was injected into the same DG at different time points after retroviral labelling. Through the interaction between EnvA viral glycoprotein and its cognate receptor, TVA, pseudotyped rabies virus can selectively infect new GCs. EnvA-ΔG-MCh rabies virus is then complemented with Rgp provided by RV-SYN-GTRgp in the new neurons and crosses synapses, labelling first-order presynaptic neurons with mCherry. Because of the absence of Rgp in traced cells, this virus will not spread any further [9] , [10] , [11] . Here we reveal the direct inputs that innervate newborn GCs over time (21, 30, 60 and 90h days post injection ( d.p.i.)). Retrograde tracing showed that the newborn GCs received afferents from intra-hippocampal cells (consisting of mature GCs, mossy cells, interneurons and area CA3 pyramidal cells), from the septum, and from the perirhinal (PRH)/lateral entorhinal cortex (LEC) (cortical layers II/III). Of these cell populations, mature GCs were a major transient input at 21–30 d.p.i., whereas innervation from interneurons, mossy cells and PRH/LEC increased over time. Patch-clamp recordings supported LEC innervation. Furthermore, mice with excitotoxic PRH/LEC lesions displayed impaired fine pattern separation ability, supporting a functional role for the connectivity between this input and new neurons. Development and validation of the dual-virus tracing system Retrograde tracers such as fluorogold label afferents [12] , albeit without selectivity or ability to cross synapses ( Supplementary Fig. S1 ). In the present experiments, we used selective rabies virus-mediated retrograde tracing originating from 'starter' cells that were pre-labelled with a Maloney murine leukaemia virus (MMLV)-based retroviral vector, to target newly born neurons [13] or pre-labelled with lentivirus, which infects both mature and immature cells [14] , [15] . To establish and test the dual-virus system in vivo , initially we used lentivirus to label 'starter' neurons with high efficiency. In particular, lentivirus, LV-SYNP-HTG (LVV) [11] , [16] , expressing TVA, Rgp and histone-tagged GFP (hGFP), was injected into the DG ( n =3). Ten days after lentivirus administration, EnvA-ΔG-MCh rabies virus (MCh) was injected into the DG to specifically infect the TVA-expressing 'starter' cells. After waiting 1 week, a time period similar to previous studies [10] , [11] , [17] , to allow the G-deleted rabies virus to complement with Rgp expressed in 'starter' cells, and spread trans-synaptically to their presynaptic projecting partners, mice were perfused and analysed histologically. Expression of MCh revealed retrograde tracing from 'starter' DG cells to local inhibitory interneurons, mossy cells, septum, medial entorhinal cortex (MEC), LEC and a 'back projection' from area CA3 (ref. 18 ) ( Fig. 1a–c ; Supplementary Fig. S1 ). Lentivirus also labelled hilar cells, which may receive area CA3 'back projections' [18] . 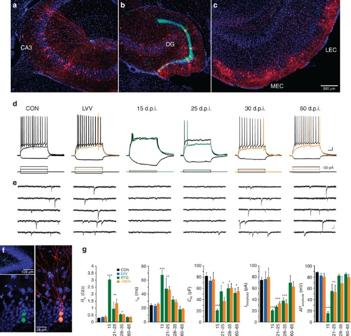Figure 1: Retrograde tracing and electrophysiological analysis of single- or dual-virus labelled GCs. Horizontal sections through (a) area CA3, (b) DG and (c) MEC and LEC, derived from a mouse injected with LVV followed by EnvA-ΔG-MCh rabies virus (red) infection Scale bar, 200 μm. (a) MCh+-labelling of area CA3 pyramidal cells. (b) hGFP+GC nuclei labelled with LVV (green). Rabies virus injected in the same location resulted in dual-labelled 'starter' cells (co-localization of green and red). (c) Afferent input from the LEC and MEC to the 'starter' cells in DG. Nuclei were labelled with 4′-6-diaminodino-2-phenylindole (DAPI) (blue). (d) Traces representative of membrane potentials in response to current injections, from newborn GCs (RTG) at different time points (15, 25, 30 and 60 d.p.i., as indicated at the top), mature unlabelled GCs (CON) and cells labelled with LVV. Recordings were made from cells with single (green trace) and double labelling (orange trace). Depolarizing steps were delivered at threshold and twice threshold current. Scale: 10 mV, 50 ms. (e) Traces representative of spontaneous postsynaptic currents recorded under voltage clamp (Vh=−80 mV; scale 10 pA, 100 ms). (f) Photomicrographs showing newborn GCs labelled with retrovirus (RTG) expressing nuclear hGFP, and MCh at 30 d.p.i. Scale bar, 25 μm. (g) Summary histograms of passive and active membrane properties. Measurements did not show significant differences between single and double labelling (P>0.05). Differences between mature and newborn GCs were analysed with Kruskal–Wallis test followed by Dunn's test, ***P<0.001, **P<0.01, *P<0.05; CON (n=20), LVV (n=8), LVV+MCh (n=5), 15 d.p.i. RTG (n=7), 21–25 d.p.i. RTG (n=3), 21–25 d.p.i. RTG+MCh (n=4), 28–35 d.p.i. RTG (n=7), 28–35 d.p.i. RTG+MCh (n=3), 60–65 d.p.i. RTG (n=3), 60–65 d.p.i. RTG+MCh (n=3). Data are means±s.e.m. DG, Dentate Gyrus; MEC, medial entorhinal cortex; LEC, lateral entorhinal cortex. Figure 1: Retrograde tracing and electrophysiological analysis of single- or dual-virus labelled GCs. Horizontal sections through ( a ) area CA3, ( b ) DG and ( c ) MEC and LEC, derived from a mouse injected with LVV followed by EnvA-ΔG-MCh rabies virus (red) infection Scale bar, 200 μm. ( a ) MCh + -labelling of area CA3 pyramidal cells. ( b ) hGFP + GC nuclei labelled with LVV (green). Rabies virus injected in the same location resulted in dual-labelled 'starter' cells (co-localization of green and red). ( c ) Afferent input from the LEC and MEC to the 'starter' cells in DG. Nuclei were labelled with 4′-6-diaminodino-2-phenylindole (DAPI) (blue). ( d ) Traces representative of membrane potentials in response to current injections, from newborn GCs (RTG) at different time points (15, 25, 30 and 60 d.p.i., as indicated at the top), mature unlabelled GCs (CON) and cells labelled with LVV. Recordings were made from cells with single (green trace) and double labelling (orange trace). Depolarizing steps were delivered at threshold and twice threshold current. Scale: 10 mV, 50 ms. ( e ) Traces representative of spontaneous postsynaptic currents recorded under voltage clamp (Vh=−80 mV; scale 10 pA, 100 ms). ( f ) Photomicrographs showing newborn GCs labelled with retrovirus (RTG) expressing nuclear hGFP, and MCh at 30 d.p.i. Scale bar, 25 μm. ( g ) Summary histograms of passive and active membrane properties. Measurements did not show significant differences between single and double labelling ( P >0.05). Differences between mature and newborn GCs were analysed with Kruskal–Wallis test followed by Dunn's test, *** P <0.001, ** P <0.01, * P <0.05; CON ( n =20), LVV ( n =8), LVV+MCh ( n =5), 15 d.p.i. RTG ( n =7), 21–25 d.p.i. RTG ( n =3), 21–25 d.p.i. RTG+MCh ( n =4), 28–35 d.p.i. RTG ( n =7), 28–35 d.p.i. RTG+MCh ( n =3), 60–65 d.p.i. RTG ( n =3), 60–65 d.p.i. RTG+MCh ( n =3). Data are means±s.e.m. DG, Dentate Gyrus; MEC, medial entorhinal cortex; LEC, lateral entorhinal cortex. Full size image We validated our strategy by using a control lentivirus LV-SYNP-HT missing Rgp, which is required for trans-synaptic spread [9] , [10] , [11] , followed by EnvA-ΔG-MCh rabies virus infection ( n =5). Only hGFP- and hGFP-MCh-expressing cells were observed ( Supplementary Fig. S2a ). Thus, in the absence of Rgp, rabies virus infected the TVA-expressing 'starter' neurons exclusively, but failed to spread beyond the initially infected cells. These findings indicate that our system is specific and efficient in vivo. Additional mice ( n =5) were injected with LVV followed by EnvA-ΔG-MCh rabies virus, and acute brain slices were prepared for patch clamp recordings from DG cells with single (hGFP) or double labelling (hGFP and MCh). Labelled cells showed active and passive membrane properties, such as resting membrane potential (RMP), input resistance ( R in ), time constant ( τ m ), membrane capacitance ( C m ), threshold current ( I threshold ), action potential (AP) amplitude, similar to control unlabelled GCs ( Fig. 1d,g ; Supplementary Table S1 ). Spontaneous postsynaptic activity was comparable to control GCs ( Fig. 1e ; Supplementary Table S1 ), suggesting no modifications in functional synaptic inputs. Thus, dual-virus infection does not modify the physiology of GCs and results in efficient retrograde labelling. Definition of time points for retrograde tracing of new GCs Before tracing inputs to newborn neurons, we first identified time points when new GCs were likely to receive functional inputs. Newborn neurons were labelled by injection of a MMLV retrovirus [13] RV-SYN-GTRgp, expressing nucleus-localized hGFP, TVA receptor and Rgp, under control of the neuron-specific synapsin promoter (RTG; Fig. 1f ). hGFP + cells expressed the immature neuronal marker doublecortin (DCX) at 15 d.p.i., further confirming the specificity of retrovirus-mediated gene transduction in newborn GCs. In addition these cells also expressed the TVA receptor ( Supplementary Fig. S3 ). At 15–25 d.p.i., acute brain slices were prepared for intracellular recordings from hGFP + neurons [13] . At 15 d.p.i. ( n =7) and 21–25 d.p.i. ( n =7), hGFP + neurons were localized in the inner GC layer of the DG and displayed passive and active membrane properties characteristic of newborn GCs [3] , [13] , [19] such as a large R in , a slower τ m , a smaller C m and more depolarized RMP compared with mature GCs ( Fig. 1d,g ; Supplementary Table S1 ). Depolarizing current injection elicited few APs with a small amplitude at low I threshold ( Fig. 1d,g ). Spontaneous postsynaptic activity was observed from 21–25 d.p.i. ( Fig. 1e ) consistent with the notion of afferent connectivity and in agreement with previous observations [19] . Therefore, the first time point chosen for retrograde tracing was 21 d.p.i. followed 1 week later by EnvA-ΔG-MCh injection (21d RTG+7d EnvA-ΔG-MCh). Subsequently, tissue from mice with dual-virus injections ( n= 4–6 mice per time point) was evaluated at 30 d.p.i. (30d RTG+7d EnvA-ΔG-MCh), 60 d.p.i. (60d RTG+7d EnvA-ΔG-MCh) and 90 d.p.i. (90d RTG+7d EnvA-ΔG-MCh). Developing GC physiology was unaffected by dual-virus labelling ( Fig. 1d,e,g ; Supplementary Table S1 ), showing properties consistent with retroviral labelling only [13] , [19] . Histological analysis showed that the number of retrovirally labelled newborn cells (hGFP + cells; F (3,15) =0.68, P >0.58), the number of newborn 'starter' cells (hGFP + -MCh + cells; F (3,15) =2.36, P >0.11) and the total number of traced cells (MCh + only) remained constant ( F (3,15) =0.52, P >0.67; Fig. 2d,e ). However, the ratio of traced cells to newborn 'starter' cells increased significantly over time ((~1:1 at 21 d.p.i. versus ~16:1 at 90 d.p.i. ); One-way analysis of variance (ANOVA), 21 d.p.i. ( n =4), 30 d.p.i. ( n =6), 60 d.p.i. ( n =4), 90 d.p.i. ( n =5); F (3,15) =5.34, P <0.01; Fig. 2f )). Thus, pre-synaptic contacts of newborn GCs increased over time throughout the brain. 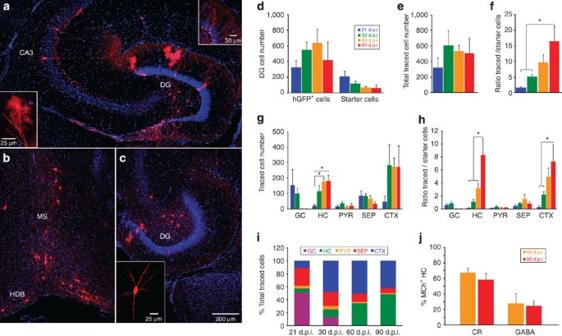Figure 2: Septal-hippocampal inputs and quantification of traced cells. (a) Horizontal section through the DG and area CA3 at 30 d.p.i. Newborn 'starter' cells express nuclear hGFP (green) and MCh (red). Trans-synaptic rabies-virus-mediated labelling (red) was observed in area CA3 pyramidal cells suggesting a direct 'back projection' to DG. Newborn neurons receive input from mature GCs (right inset, scale bar, 50 μm). Astrocytes surrounded the dendritic arborization of newborn 'starter' cells (left inset, scale bar 25 μm). (b) Traced cells labelled with MCh in the medial septum (MS) and horizontal nucleus of the diagonal band (HDB) at 21 d.p.i. (coronal section). (c) MCh+- HC at 30 d.p.i. (horizontal section) and a characteristic mossy cell (inset, scale bar, 25 μm). Overview panelsa,b,c, scale bar, 200 μm. Nuclei are labelled with DAPI (blue). (d–j) Quantification and characterization of afferent input to newborn GCs. (d) hGFP+new GCs and, starter cells (dual-labelled hGFP+-MCh+new GCs), remained stable over time. (e) The total number of traced cells did not differ across time points. (f) The ratio of traced to 'starter' cells was significantly increased at 90 d.p.i compared with 21 d.p.i. and 30 d.p.i., suggesting a strengthening of inputs to new GCs. (g) Upon evaluation across time points and brain regions a transient input from mature to newborn GCs was observed, whereas hilar afferents increased significantly compared to 21 d.p.i. (h) The ratio of traced HC to 'starter' cells was increased significantly at 90 d.p.i. compared with all other time points. Similarly, distal cortical input differed from 21 d.p.i. and 30 d.p.i. at 90 d.p.i. (i) Percentage input from mature GC was high at 21 d.p.i. but was absent at 60 and 90 d.p.i. Both hilar (60 d.p.i. and 90 d.p.i. versus 21 d.p.i. and 30 d.p.i.) and distal cortical (30, 60, 90 d.p.i. versus 21 d.p.i.) inputs increased over time. The septal and area CA3 cells remained stable over time. (j) Quantification of intra-hippocampal MCh+cells double labelled with calretinin (CR), a marker for mossy cells, or GABA, a marker for inhibitory interneurons, at 60 d.p.i. and 90 d.p.i. *P<0.05, One-way ANOVA followed by Fisher's post-hoct-tests, 21 d.p.i. (n=4), 30 d.p.i. (n=6), 60 d.p.i. (n=4), 90 d.p.i. (n=5). Data are means±s.e.m. HC, hilar cells; GC, granule cells; PYR, area CA3 pyramidal cells; SEP, septal cells; CTX, cortical cells. Figure 2: Septal-hippocampal inputs and quantification of traced cells. ( a ) Horizontal section through the DG and area CA3 at 30 d.p.i. Newborn 'starter' cells express nuclear hGFP (green) and MCh (red). Trans-synaptic rabies-virus-mediated labelling (red) was observed in area CA3 pyramidal cells suggesting a direct 'back projection' to DG. Newborn neurons receive input from mature GCs (right inset, scale bar, 50 μm). Astrocytes surrounded the dendritic arborization of newborn 'starter' cells (left inset, scale bar 25 μm). ( b ) Traced cells labelled with MCh in the medial septum (MS) and horizontal nucleus of the diagonal band (HDB) at 21 d.p.i. (coronal section). ( c ) MCh + - HC at 30 d.p.i. (horizontal section) and a characteristic mossy cell (inset, scale bar, 25 μm). Overview panels a , b , c , scale bar, 200 μm. Nuclei are labelled with DAPI (blue). ( d – j ) Quantification and characterization of afferent input to newborn GCs. ( d ) hGFP + new GCs and, starter cells (dual-labelled hGFP + -MCh + new GCs), remained stable over time. ( e ) The total number of traced cells did not differ across time points. ( f ) The ratio of traced to 'starter' cells was significantly increased at 90 d.p.i compared with 21 d.p.i. and 30 d.p.i., suggesting a strengthening of inputs to new GCs. ( g ) Upon evaluation across time points and brain regions a transient input from mature to newborn GCs was observed, whereas hilar afferents increased significantly compared to 21 d.p.i. ( h ) The ratio of traced HC to 'starter' cells was increased significantly at 90 d.p.i. compared with all other time points. Similarly, distal cortical input differed from 21 d.p.i. and 30 d.p.i. at 90 d.p.i. ( i ) Percentage input from mature GC was high at 21 d.p.i. but was absent at 60 and 90 d.p.i. Both hilar (60 d.p.i. and 90 d.p.i. versus 21 d.p.i. and 30 d.p.i.) and distal cortical (30, 60, 90 d.p.i. versus 21 d.p.i.) inputs increased over time. The septal and area CA3 cells remained stable over time. ( j ) Quantification of intra-hippocampal MCh + cells double labelled with calretinin (CR), a marker for mossy cells, or GABA, a marker for inhibitory interneurons, at 60 d.p.i. and 90 d.p.i. * P <0.05, One-way ANOVA followed by Fisher's post-hoc t -tests, 21 d.p.i. ( n =4), 30 d.p.i. ( n =6), 60 d.p.i. ( n =4), 90 d.p.i. ( n =5). Data are means±s.e.m. HC, hilar cells; GC, granule cells; PYR, area CA3 pyramidal cells; SEP, septal cells; CTX, cortical cells. Full size image We validated retrograde tracing of newborn GCs by using RV-SYN-HT missing Rgp (21 d.p.i.) followed by EnvA-ΔG-MCh rabies virus injection ( n =3). No viral spread beyond the initially infected cells was observed ( Supplementary Fig. S2b ). Furthermore, injection of EnvA-ΔG-MCh rabies virus only did not infect any cells, indicating that the entry of our rabies virus into 'starter' cells is dependent on the TVA receptor ( Supplementary Fig. S4 ). Intra-hippocampal inputs to newborn GCs Our approach identified several intra-hippocampal afferents to new GCs. Transient input from mature GCs to new neurons was observed in the first month after viral labelling. In addition, hilar cell (HC; interneurons and mossy cells) innervation increased over time. Furthermore, connectivity from area CA3 pyramidal cells was detected at all time points investigated. Altogether these hippocampal cells provide a local network of innervation to newborn GCs ( Figs 2a,c and 3 , Supplementary Fig. S5 ). 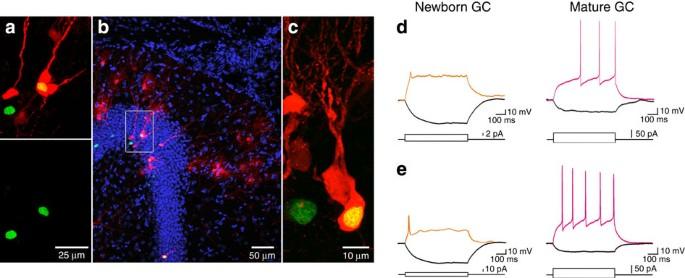Figure 3: Mature GCs provide input to new neurons in the DG. (a) Photomicrograph showing newborn cells (30 d.p.i.) expressing nuclear hGFP (green nucleus) only or both hGFP and cytoplasmic MCh (yellow nucleus, 'starter' cell) and mature traced GCs expressing MCh (red) only Scale bar, 25μm. (b) Overview of the horizontal section that includes the cells shown in (a), boxed. Nuclei are labelled with DAPI (blue) Scale bar, 50μm. (c) An additional example of the close association between a mature MCh+traced cell (red) and a newborn 'starter cell' (red+green=yellow nucleus) Scale bar, 10μm. (d,e) Representative patch-clamp recordings from cells with dual labelling (hGFP++ and MCh+) and cells expressing only MCh at short intervals after virus injections Scale bar, 10μm. (d) 7 d.p.i (7d RTG+6d EnvA-ΔG-MCh+). (e) 14 d.p.i (14d RTG+6d EnvA-ΔG-MCh). Cells co-expressing hGFP and MCh (orange traces) show physiological properties of immature newborn GCs. Cells expressing MCh only (pink traces) show properties of mature GCs. Recordings were obtained from the same slice at each time point. Figure 3: Mature GCs provide input to new neurons in the DG. ( a ) Photomicrograph showing newborn cells (30 d.p.i.) expressing nuclear hGFP (green nucleus) only or both hGFP and cytoplasmic MCh (yellow nucleus, 'starter' cell) and mature traced GCs expressing MCh (red) only Scale bar, 25μm. ( b ) Overview of the horizontal section that includes the cells shown in ( a ), boxed. Nuclei are labelled with DAPI (blue) Scale bar, 50μm. ( c ) An additional example of the close association between a mature MCh + traced cell (red) and a newborn 'starter cell' (red+green=yellow nucleus) Scale bar, 10μm. ( d , e ) Representative patch-clamp recordings from cells with dual labelling (hGFP + + and MCh+) and cells expressing only MCh at short intervals after virus injections Scale bar, 10μm. ( d ) 7 d.p.i (7d RTG+6d EnvA-ΔG-MCh + ). ( e ) 14 d.p.i (14d RTG+6d EnvA-ΔG-MCh). Cells co-expressing hGFP and MCh (orange traces) show physiological properties of immature newborn GCs. Cells expressing MCh only (pink traces) show properties of mature GCs. Recordings were obtained from the same slice at each time point. Full size image Analysis of MCh + cells revealed retrograde tracing of mature GCs (MCh + only) at 21 and 30 d.p.i., suggesting a local connectivity between mature and newborn GC ( Fig. 3a–c ). To rule out the possibility that cells expressing only MCh were in fact newborn GCs with low expression of hGFP, we performed intracellular recordings from cells with dual labelling (hGFP-MCh) and cells expressing MCh only at short intervals after virus injections (7 d.p.i. (7d RTG+6d EnvA-ΔG-MCh) and 14 d.p.i. (14d RTG+6d EnvA-ΔG-MCh)). At these time points, young dual-labelled (hGFP-MCh) GCs had immature physiological properties, whereas cells expressing only MCh showed mature GC characteristics, in the same acute slice preparation ( Fig. 3d,e ). Quantification of GCs expressing only MCh showed that these cells represented 51±21.2% ( n =4) of total traced cell number at 21 d.p.i., however, at 30 d.p.i., the percentage decreased to 15±2.5% ( n =6) and they were no longer observed at 60 d.p.i. ( Fig. 2g-i ). Thus, our results suggest a substantial but transient synaptic connectivity between young and mature GCs. Retrograde tracing revealed local innervation from HC (interneurons and mossy cells) ( Figs 2c and 4a,c–f ). Quantification of the number of HC revealed a significant increase at 60 d.p.i. (177±24 cells) and 90 d.p.i. (180±36 cells) as compared with 21 d.p.i. (18±7 cells), ((One-way ANOVA, 21 d.p.i. ( n =4), 30 d.p.i. ( n =6), 60 d.p.i. ( n =4), 90 d.p.i. ( n =5); F (3,15) =4.72, P <0.02; Fig. 2g )). Ratio of MCh + HC to newborn 'starter' cells increased significantly from ~3:1 to ~8:1 at 60 and 90 d.p.i., respectively ((One-way ANOVA, 21 d.p.i. ( n =4), 30 d.p.i. ( n =6), 60 d.p.i. ( n =4), 90 d.p.i. ( n =5); F (3,15) =7.24, P <0.003; Fig. 2h )). HC represented 32.2±3.8% (60 d.p.i.) and 48.2±8.4% (90 d.p.i.) of the total traced cells ( Fig. 2i ). 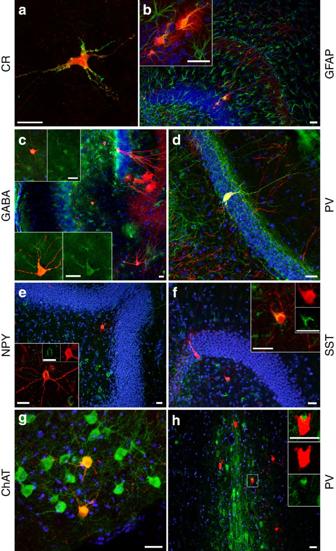Figure 4: Neurochemical characterization of cells trans-synaptically labelled with rabies virus. (a) MCh+hilar cell immunoreactive for CR, a characteristic mossy cell marker. (b) MCh+cells immunoreactive for GFAP, a marker for astrocytes. (c) GABA+-MCh+cells in the DG and CA3c with differential morphology. Top inset shows a MCh-GABA+cell with a small soma. Bottom inset shows a cell with a large soma in area CA3c. (d) Double-labelling of MCh and PV, a marker for interneurons, was observed. (e) NPY, a marker characteristic for interneurons was expressed in MCh+cells. Inset shows co-localization. (f) MCh+cell double-labelled with SST. Inset shows co-localization. (g) MCh+cells in the horizontal nucleus of the diagonal band (HDB) were immunoreactive for ChAT, coronal section. (h) No double labelling between MCh+cells and PV was observed in the medial septum (MS), coronal section. The markers are green, MCh+cells red and DAPI labelling of nuclei blue. All scale bars, 25 μm. Figure 4: Neurochemical characterization of cells trans-synaptically labelled with rabies virus. ( a ) MCh + hilar cell immunoreactive for CR, a characteristic mossy cell marker. ( b ) MCh + cells immunoreactive for GFAP, a marker for astrocytes. ( c ) GABA + -MCh + cells in the DG and CA3c with differential morphology. Top inset shows a MCh-GABA + cell with a small soma. Bottom inset shows a cell with a large soma in area CA3c. ( d ) Double-labelling of MCh and PV, a marker for interneurons, was observed. ( e ) NPY, a marker characteristic for interneurons was expressed in MCh + cells. Inset shows co-localization. ( f ) MCh + cell double-labelled with SST. Inset shows co-localization. ( g ) MCh + cells in the horizontal nucleus of the diagonal band (HDB) were immunoreactive for ChAT, coronal section. ( h ) No double labelling between MCh + cells and PV was observed in the medial septum (MS), coronal section. The markers are green, MCh + cells red and DAPI labelling of nuclei blue. All scale bars, 25 μm. Full size image Neurochemical characterization of MCh + HC showed that 67.1±5.9% (60 d.p.i. ; n =4) and 57.6±8.7% (90 d.p.i. ; n =5) of these cells are immunoreactive for calretinin (CR), a marker for most mossy cells [20] ( Figs 2j and 4a ). These cells had characteristic thorny excrescences and were localized in the hilus ( Figs 2c and 4a ). GABA immunoreactivity was observed in 27.6±12.4% (60 d.p.i.) and 24.6±6.5% (90 d.p.i.) of the MCh + cells ( Figs 2j and 4c ). GABA + -MCh + cells were observed in the hilus, molecular layer of the DG and area CA3c. Characteristic markers of GABAergic interneurons, such as parvalbumin (PV), neuropeptide Y (NPY) and somatostatin (SST) were also evaluated. PV + -MCh + immunoreactivity was observed in 17.7±9.2% (60 d.p.i.) and 12.1±4.7% (90 d.p.i.) of the MCh + cells ( Fig. 4d ). NPY was expressed in 11.9±6.1% (60 d.p.i.) and 20.4±8.7% (90 d.p.i.) of the MCh + cells ( Fig. 4e ). SST was expressed in 13.4±3.3% (60 d.p.i.) and 16.4±7.4% (90 d.p.i.) of the MCh + cells ( Fig. 4f ). It should be noted that SST + interneurons can co-express NPY [21] . A direct 'back projection' from CA3 pyramidal cells to newborn GCs was observed at all time points ( Fig. 2a,g–i , Supplementary Fig. S5 ). Quantification of MCh + CA3 pyramidal cells showed a rather sparse but stable number of cells over time ( Fig. 2g,h ). These cells represented less than 10% of the total traced cells ( Fig. 2i ). Interestingly, MCh + cells with glial characteristics were closely associated with the dendrites/spines of new GCs ( Fig. 2a left inset). Patch-clamp recordings indicated that these cells do not fire APs (RMP=−73.5±1.5 mV; R in =189±7 MΩ; C m =50.5±1.5 pF; n =2), and double labelling for GFAP suggested that they are astrocytes ( Fig. 4b ). Analysis of the ratio of these astrocytes to newborn 'starter' cells revealed a significant increase at 60 d.p.i. (~3:1) and 90 d.p.i. (~3:1) as compared with 21 d.p.i. (~1:10), when very few astrocytes were associated with 'starter' cells ((one-way ANOVA, 21 d.p.i. ( n =3), 30 d.p.i. ( n =3), 60 d.p.i. ( n =4), 90 d.p.i. ( n =5); F (3,11) =3.71, P <0.04)). Interestingly, the temporal appearance of these astrocytes corresponds with the observed increase in innervation of new neurons as they mature. These cells may enhance new neuron integration through synapse-like contacts with new GCs [22] . Distal subcortical areas innervate newborn GCs Retrograde tracing showed robust and stable inputs over time from the septum and horizontal nucleus of the diagonal band of Broca ( Fig. 2b,g–i ); areas characterized by the presence of cholinergic and PV-immunoreactive GABAergic neurons [23] . To investigate the identity of MCh + cells in the septum, we performed immunostaining for choline-acetyltransferase (ChAT), a marker for cholinergic neurons, and PV. We observed consistent double labelling of MCh + cells with ChAT but not with PV, suggesting that septal input to newborn GCs is cholinergic ( Fig. 4g,h ). Retrograde tracing also showed afferents originating from the mammillary bodies ( Supplementary Fig. S6 ). Distal cortical input to the newborn GCs The entorhinal cortex (EC) provides the hippocampus with its major excitatory glutamatergic input from the MEC and LEC through the medial (MPP) and lateral (LPP) perforant pathway, coursing through the medial (M-ML) and outer molecular layer (O-ML), respectively [24] . Retrograde tracing showed cortical labelling (CTX) mainly in layers II and III of the PRH and LEC ( Figs 5a–c and 6 ; Supplementary Figs S1p–t and Supplementary Fig. S7 ), and sparsely in the dorsal caudal-medial entorhinal cortex (CEnt), ( Fig. 6b , Supplementary Fig. S8 ). Labelling increased after 21 d.p.i. (45±37 cells ( n =4)), and became robust over time (273±58 cells (60 d.p.i. ; n =4)) ( Fig. 2g ). Ratio of CTX MCh + cells to newborn 'starter' cells increased significantly from ~2:1 at 30 d.p.i. to ~7:1 at 90 d.p.i. ((one-way ANOVA, 21 d.p.i. ( n =4), 30 d.p.i. ( n =6), 60 d.p.i. ( n =4), 90 d.p.i. ( n =5); F (3,15) =4.09, P <0.03; Fig. 2h )) and became a major afferent to the newborn GCs (>40% of the total number of traced cells) from 30 d.p.i. ((one-way ANOVA, 21 d.p.i. ( n =4), 30 d.p.i. ( n =6), 60 d.p.i. ( n =4), 90 d.p.i. ( n =5); F (3,15) =4.32, P <0.02; Fig. 2i )) with axons localized in the O-ML ( Figs 5d and 6 ). 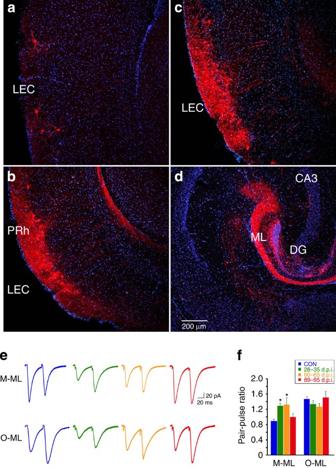Figure 5: LEC input mediated synaptic plasticity of newborn GCs. (a,b,c) Horizontal sections showing confocal images of trans-synaptic labelling (MCh, red) in the EC at (a) 21 d.p.i. (b) 30 d.p.i. (c) 60 d.p.i. (d) Photomicrograph of the perforant pathway innervating mainly the O-ML of the DG at 90 d.p.i. Scale bar, 200 μm. (e) Representative traces of pairs of EPSCs evoked at 50 ms of inter-pulse intervals by stimulation of the O-ML and M-ML in mature control cells (n=8) and newborn GCs at 28–35 d.p.i. (n=6), 60–65 d.p.i. (n=5) and 89–95 d.p.i. (n=6), colour code matches the graph inf. (f) Comparison of the paired-pulse ratio (EPSC2/EPSC1) of EPSCs evoked at 50 ms inter-pulse intervals (left). *P<0.05, Student'st-test, mature control cells (n=8); newborn GCs: 28–35 d.p.i (n=6), 60–65 d.p.i. (n=5) and 89–95 d.p.i. (n=6). Data are means±s.e.m. Nuclei are DAPI (blue). DG, Dentate gyrus; LEC, lateral entorhinal cortex; PRh, perirhinal cortex; ML, molecular Layer; CA3, area CA3. Figure 5: LEC input mediated synaptic plasticity of newborn GCs. ( a , b , c ) Horizontal sections showing confocal images of trans-synaptic labelling (MCh, red) in the EC at ( a ) 21 d.p.i. ( b ) 30 d.p.i. ( c ) 60 d.p.i. ( d ) Photomicrograph of the perforant pathway innervating mainly the O-ML of the DG at 90 d.p.i. Scale bar, 200 μm. ( e ) Representative traces of pairs of EPSCs evoked at 50 ms of inter-pulse intervals by stimulation of the O-ML and M-ML in mature control cells ( n =8) and newborn GCs at 28–35 d.p.i. ( n =6), 60–65 d.p.i. ( n =5) and 89–95 d.p.i. ( n =6), colour code matches the graph in f . ( f ) Comparison of the paired-pulse ratio (EPSC2/EPSC1) of EPSCs evoked at 50 ms inter-pulse intervals (left). * P <0.05, Student's t -test, mature control cells ( n =8); newborn GCs: 28–35 d.p.i ( n =6), 60–65 d.p.i. ( n =5) and 89–95 d.p.i. ( n =6). Data are means±s.e.m. Nuclei are DAPI (blue). DG, Dentate gyrus; LEC, lateral entorhinal cortex; PRh, perirhinal cortex; ML, molecular Layer; CA3, area CA3. 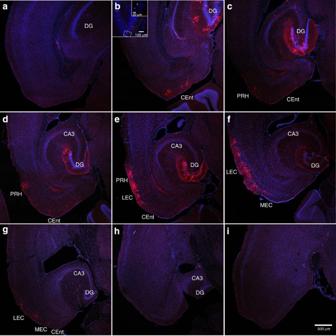Figure 6: Overview of the retrograde tracing pattern to newborn 'starter' GCs at 90 d.p.i. (a–i) Equidistant horizontal sections (480 μm between each section) were imaged at low power (×4 objective) throughout the dorsal-ventral extent of the hippocampus and adjacent cortex. Scale bar, 500 μm. (b–g) Trans-synaptic rabies-virus-mediated labelling (MCh, red) was observed mainly in PRH and LEC. (b) Inset shows hGFP+-MCh+newborn GCs in DG. Scale bars, 20 μm and 100 μm. Nuclei are labelled with DAPI (blue). CEnt, caudal medial entorhinal cortex; LEC, lateral entorhinal cortex; MEC, medial entorhinal cortex; PRH, perirhinal cortex. Full size image Figure 6: Overview of the retrograde tracing pattern to newborn 'starter' GCs at 90 d.p.i. ( a – i ) Equidistant horizontal sections (480 μm between each section) were imaged at low power (×4 objective) throughout the dorsal-ventral extent of the hippocampus and adjacent cortex. Scale bar, 500 μm. ( b – g ) Trans-synaptic rabies-virus-mediated labelling (MCh, red) was observed mainly in PRH and LEC. ( b ) Inset shows hGFP + -MCh + newborn GCs in DG. Scale bars, 20 μm and 100 μm. Nuclei are labelled with DAPI (blue). CEnt, caudal medial entorhinal cortex; LEC, lateral entorhinal cortex; MEC, medial entorhinal cortex; PRH, perirhinal cortex. Full size image To physiologically examine the time course of afferent innervation from EC, we performed patch-clamp recordings from mature and newborn GCs at different developmental stages. Short-term synaptic plasticity was evaluated by paired-pulse stimulation at 50 ms inter-pulse intervals delivered to O-ML or M-ML. Stimulation of O-ML evoked paired-pulse facilitation, characteristic of LEC input [25] in mature and newborn GCs at all the time points ( Fig. 5e,f ). M-ML stimulation revealed paired-pulse depression in mature GCs ( n =8), characteristic of MEC input [25] . In contrast, newborn GCs displayed paired-pulse facilitation at 28–35 d.p.i. ( n =6) and 60–65 d.p.i. ( n =5). Only a modest paired-pulse depression was observed at 90 d.p.i. ( n =6) ( Fig. 5e,f ). To further examine the selectivity of the synaptic input onto the newborn GCs, excitotoxic MEC or LEC lesions were performed and the synaptic response to stimulation of the MPP and LPP was analysed. MEC lesions did not change the response evoked in newborn GCs at 30 d.p.i. However, LEC lesion resulted in a reduced synaptic response evoked by stimulation of the LPP but not MPP ( Supplementary Fig. S9 ). Altogether, these results suggest a differential synaptic input integration between newborn and mature GCs, consistent with previous studies [2] , [26] . To evaluate whether specific EC cell types project to newborn GCs, patch-clamp recordings of MCh + cells were performed. A total of 15 cells from LEC layer II and III were recorded ( Fig. 7a,b ). Based on passive and active membrane properties, such as R in , RMP, AP amplitude, firing frequency and sag presence, five different cell types were identified. Intrinsic properties were consistent with characteristics of putative stellate cells (Type 1; n =2; Fig. 7c ), multipolar cells, (Type II; n =2; Fig. 7d ), pyramidal cells (Type III; n= 6; Fig. 7e ) and two different types of cells with irregular firing distinguishable by sag presence (Type IV and V; n =5; Fig. 7f–i ; Supplementary Table S2 ). 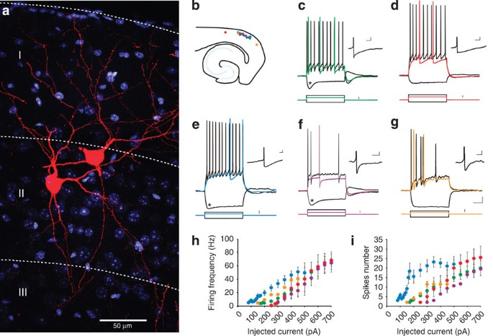Figure 7: Electrophysiological characterization of LEC cells projecting to newborn GCs. (a) Photomicrograph showing MCh+-putative multipolar neurons in LEC layer II. Nuclei are labelled with DAPI (blue). Scale bar, 50 μm. (b) Schematic representation of the location of MCh+-recorded cells; different types of cells are represented by the respective colours in (c–g) Representative traces of membrane potential changes in response to current injection of a putative stellate cell (c; Type I), pyramidal cell (d; Type II), multipolar cell (e; Type III) and two different types of cells with irregular firing differentiated by sag presence (fandg; Type IV and V, respectively). Prominent sag (onset indicated by asterisk) was present in some cell types at hyperpolarization. Depolarizing steps were delivered to threshold and twice-threshold current. Scale 10 mV, 50 ms. Insets show enlarged spike after-potentials. Scale: 5 mV, 5 ms. (h) Differential firing frequency in response to increasing current steps of the different types of cells. (i) Number of spikes elicited at different current steps. Type I,n=2 (green), Type II,n=2 (red), Type III,n=6 (blue), Type IV,n=3 (purple) and Type V,n=2 (orange). Data are means±s.e.m. Figure 7: Electrophysiological characterization of LEC cells projecting to newborn GCs. ( a ) Photomicrograph showing MCh + -putative multipolar neurons in LEC layer II. Nuclei are labelled with DAPI (blue). Scale bar, 50 μm. ( b ) Schematic representation of the location of MCh + -recorded cells; different types of cells are represented by the respective colours in ( c – g ) Representative traces of membrane potential changes in response to current injection of a putative stellate cell ( c ; Type I), pyramidal cell ( d ; Type II), multipolar cell ( e ; Type III) and two different types of cells with irregular firing differentiated by sag presence ( f and g ; Type IV and V, respectively). Prominent sag (onset indicated by asterisk) was present in some cell types at hyperpolarization. Depolarizing steps were delivered to threshold and twice-threshold current. Scale 10 mV, 50 ms. Insets show enlarged spike after-potentials. Scale: 5 mV, 5 ms. ( h ) Differential firing frequency in response to increasing current steps of the different types of cells. ( i ) Number of spikes elicited at different current steps. Type I, n =2 (green), Type II, n =2 (red), Type III, n =6 (blue), Type IV, n =3 (purple) and Type V, n =2 (orange). Data are means±s.e.m. Full size image Lesion of PRH/LEC input impairs spatial pattern separation The functional significance of the PRH/LEC input to newborn neurons was evaluated in behavioural tests: spatial pattern separation in the touchscreen system to test DG function [6] , [27] , and a hippocampus-dependent task, the Morris water maze [28] . After 1 month of shaping to the touchscreen task, mice were systemically injected with BrdU over 6 days ( Supplementary Fig. S10 ; Supplementary methods ) and then underwent bilateral PRH/LEC infusion with phosphate-buffered saline (PBS) ( n =16) or N -methyl- D -aspartate (NMDA) ( n =10). Subsequently, mice underwent task training with an intermediate separation between stimuli on the touchscreen [27] . The average number of days to complete the task training did not differ between groups (PBS: 4.5±0.22 days; NMDA: 4.8±0.42 days; t (24) =0.69, P >0.49), nor did the trials to criterion ( F (1,24) =0.99, P >0.33). After task training, mice were tested in probe trials with either small or big separations between the stimuli ( Fig. 8a ). Analysis of trials to criterion revealed a significant interaction between group and separation ((ANOVA with repeated measures, PBS ( n =16), NMDA ( n =10), F (1,24) =9.97, P <0.004)), and a significant main effect of separation ( F (1,24) =37.1, P <0.0001). Post-hoc comparisons revealed a significant difference between PBS and NMDA groups for the small separation ((Fisher's two-tailed independent sample t -test, PBS ( n =16), NMDA ( n =10), P <0.01)) but not the big separation ( P >0.87). Subsequent testing in the Morris water maze over 5 days revealed no differences between groups in acquisition ( F (1,24) =0.08, P =0.78; Fig. 8b ) or retention of the task in a probe trial 4 h after the last training trial on day 5 ((one-way ANOVA over quadrants within groups, PBS ( n =16), F (3,60) =10.11, P <0.0001; NMDA, ( n =10) F (3,36) =4.31, P <0.01; Fig. 8c )). No difference in swim speed ( F (1,24) =0.21, P >0.65) or in latency to reach the visible platform ( t (24) =0.34, P =0.74) between groups was observed. Histological analysis showed no change in DG neurogenesis ( Supplementary Fig. S10 ) and that the lesions were restricted to the PRH/LEC ( Fig. 8d,e ). 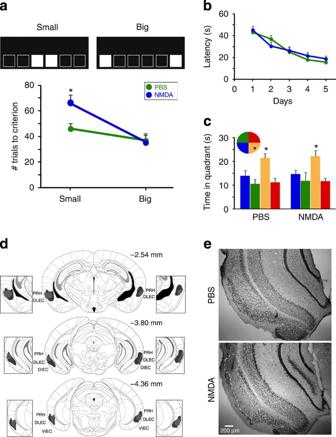Figure 8: Excitotoxic PRH/LEC lesion impairs spatial pattern separation. (a) The touchscreen paradigm acquisition of big and small separation between stimuli, was tested in NMDA- (n=10) and PBS- (n=16) injected mice. Mice were trained to reach a criterion where seven of eight trials were performed correctly. The NMDA group showed significantly impaired performance in acquisition of the small separation condition as compared to the PBS group (*P<0.01, ANOVA, PBS (n=16), NMDA (n=10). There was no difference between groups when separation between stimuli was big (P>0.87). Data are means±s.e.m. (b) Morris water maze acquisition with four training trials per day over 5 days revealed no difference in the latency to reach the hidden platform between groups. Data are means±s.e.m. (c) Retention was assessed in a probe trial 4 h after the last training trial on day 5. Both groups showed a significant preference for the target areas as compared with all other quadrants of the pool (*P<0.01, ANOVA, PBS (n=16), NMDA (n=10)). Data are means±s.e.m. (d) Series of coronal planes (adapted from Paxinos and Franklin6058) showing reconstruction of the smallest (light grey) and largest (dark grey) extent of PRH/LEC lesion. (e) Representative photomicrographs of the PRH/LEC cortex from PBS and NMDA groups (coronal sections labelled with neuronal marker NeuN) Scale bar, 200 μm. DIEC, dorsal intermediate entorhinal cortex; DLEC, dorsolateral entorhinal cortex; VIEC, ventral intermediate entorhinal cortex. Figure 8: Excitotoxic PRH/LEC lesion impairs spatial pattern separation. ( a ) The touchscreen paradigm acquisition of big and small separation between stimuli, was tested in NMDA- ( n =10) and PBS- ( n =16) injected mice. Mice were trained to reach a criterion where seven of eight trials were performed correctly. The NMDA group showed significantly impaired performance in acquisition of the small separation condition as compared to the PBS group (* P <0.01, ANOVA, PBS ( n =16), NMDA ( n =10). There was no difference between groups when separation between stimuli was big ( P >0.87). Data are means±s.e.m. ( b ) Morris water maze acquisition with four training trials per day over 5 days revealed no difference in the latency to reach the hidden platform between groups. Data are means±s.e.m. ( c ) Retention was assessed in a probe trial 4 h after the last training trial on day 5. Both groups showed a significant preference for the target areas as compared with all other quadrants of the pool (* P <0.01, ANOVA, PBS ( n =16), NMDA ( n =10)). Data are means±s.e.m. ( d ) Series of coronal planes (adapted from Paxinos and Franklin 60 [58] ) showing reconstruction of the smallest (light grey) and largest (dark grey) extent of PRH/LEC lesion. ( e ) Representative photomicrographs of the PRH/LEC cortex from PBS and NMDA groups (coronal sections labelled with neuronal marker NeuN) Scale bar, 200 μm. DIEC, dorsal intermediate entorhinal cortex; DLEC, dorsolateral entorhinal cortex; VIEC, ventral intermediate entorhinal cortex. Full size image Identification of the direct synaptic inputs to newborn GC is essential to understanding how these cells are activated and function within the neuronal network of the adult brain. Here we show that newborn GCs receive afferents from three major brain regions important for learning and memory. These are intra-hippocampal cells consisting of HC (interneurons and mossy cells), area CA3 pyramidal cells and mature GCs; septal cholinergic cells; and distal cortex, from PRH and LEC, consistent with the role of newborn GCs in contextual memory processes. In general, the 'trisynaptic hippocampal circuit' is considered unidirectional, a pathway that relays information from EC to DG, DG to CA3 pyramidal cells and CA3 to CA1 pyramidal cells [29] . In the present study, we observed a direct 'back projection' from area CA3 to mature and new GCs. Previous anatomical and physiological studies have shown evidence of an inhibitory di-synaptic 'back projection' to DG [18] . However, our findings are consistent with anatomical studies that show that CA3 pyramidal cells labelled in vivo project axons to the GC layer that terminate in the inner molecular layer [30] , [31] . Possibly, cells other than GCs might have been labelled in the lentivirus experiments, such as mossy cells or hilar interneurons, which are known to receive 'back projections' from CA3 pyramidal cells [18] . Even so, our combined MMLV-retrovirus and rabies virus labelling study supports the notion of a direct 'back projection' from area CA3 that may be unique to newborn neurons. Indeed, a recent study suggests that area CA3 may influence new GC survival [32] . Furthermore, direct input from area CA3 to newborn GCs supports a specific role for new neurons in physiological processing of sequential memories [33] and in pattern separation [34] . Recurrent excitatory circuits between GCs have previously only been observed after EC lesion [35] or epilepsy, which can induce mossy fibre sprouting into the molecular layer [36] , [37] . However, our results show substantial connectivity between mature and newborn GCs during the first month of age under normal conditions. This input may facilitate activity-dependent maturation of new GCs mediated by NMDA receptors [38] , before the arrival of EC input. Further ultrastructural studies defining the location and type of synapses that are made between mature and young cells will provide insight into the functional significance of this connectivity. In addition to mature GCs, input from CR + mossy cells was observed at all time points. Mossy cells have been described as necessary for new GC maturation and integration [39] . Altogether, local glutamatergic innervation from mature GCs, CA3 pyramidal cells and mossy cells, as well as from GABAergic inhibitory interneurons, may regulate newborn GC dendritic maturation and circuit integration before and during the arrival of cortical input. In addition, the temporary input from mature GCs may provide a mechanistic explanation for their transiently enhanced excitability during development in the adult brain [3] , [4] . The functional contribution of new GCs to learning and memory is further supported by input from cholinergic septal cells [40] . Indeed, acetylcholine receptors are present on the somta of immature GCs [41] and their activation promotes progenitor cell proliferation in vivo [42] . Furthermore, acetylcholine may modulate the excitability of the newborn GCs by increasing their firing rate, which in turn may facilitate information output to CA3 as has been observed in mature GCs [43] . In addition to septal input, subcortical connectivity from the mammillary bodies [44] to newborn neurons was observed. This connectivity may facilitate the input from the perforant pathway [45] as well as theta rhythm generation in newborn GCs [46] . Interestingly, monoaminergic projections from the ventral tegmentum and the locus coereleus were not observed [47] , [48] . Possibly, dopaminergic and noradrenergic signalling could be mediated by diffusion-based volume transmission [49] . Indeed, afferents terminating upon rabies virus-infected neurons are ubiquitously labelled when connected by chemical synapses [17] . The LEC and PRH are considered to integrate novel environmental information [50] , [51] . Evidence of a direct input from PRH to DG has been controversial [52] , [53] , however, we show a monosynaptic connection, possibly selective for newborn GCs. PRH/LEC excitotoxic lesions modified synaptic input to new neurons. Upon behavioural testing of mice that had sustained PRH/LEC lesions, no impairment in the Morris water maze was observed, consistent with previous studies [54] , [55] . However, when the mice were tested in a pattern separation paradigm, a selective deficit was observed when the distance between identical stimuli was small. A similar impairment has been associated with the functional role of newborn GCs [6] . Here, loss of PRH/LEC input in the absence of changes in new GC number appears to disrupt the ability to make fine spatial distinctions. Indeed, PRH has been implicated in pattern separation [56] , [57] , suggesting a possible interdependence between this structure and newborn GCs. Interestingly, the PRH/LEC is one of the first brain areas affected in Alzheimer's disease [58] . Altogether, our results suggest that newborn GCs are central components of memory circuits. Future studies that consider PRH/LEC, the neurogenic DG and area CA3 circuitry as a functional unit will be needed to elucidate the significance of adult neurogenesis. Animals Male C57Bl/6 mice (Jackson Labs), 5- to 6-week-old ( n =134) were housed in standard conditions with 3–4 mice per cage with food and water available ad libitum . Animals were maintained according to the National Institutes of Health guidelines, and protocols for procedures were approved by Institutional Animal Care and Use Committees at NIA, the Salk Institute and Cleveland Clinic. Viral vector production Retrovirus and lentivirus: MMLV Retroviral (RV-SYN-GTRgp) and Lentiviral (LV-SYNP-HTG) vectors were generated to express nucleus-localized green fluorescent protein (GFP), the avian viral receptor TVA and the rabies virus glycoprotein (Rgp) under the control of synapsin promoter, each gene linked by a 'self-cleaving' peptide, 2A, derived from picornavirus [59] . In addition, retroviral and lentiviral vectors missing Rgp (RV-SYN-HT and LV-SYNP-HT, respectively), only expressing GFP and TVA were designed to validate trans-synaptic tracing. Retrovirus was produced by transient transfection of vector (7.5 μg), CMVGagPol (5 μg) and CMV-VSVG (2.5 μg) in 90% confluent 293T cells grown in 10-cm plates. Virus-containing supernatant was harvested 36 h later [13] . Similarly, lentivirus was produced by transient transfection of four plasmids: vector (7.5 μg), MDL (5 μg), RSV-REV (1.9 μg) and CMV-VSVG (2.5 μg). After 48 h, supernatant was collected, filtered and concentrated by ultracentrifugation (2×2 h at 19,400 r.p.m.) [15] . The final titres of both viruses were estimated to be ~10×E8 i.u. ml −1 as determined by infection of serially diluted virus into 293T cells. EnvA-pseudotyped Δgp-mCherry rabies virus (EnvA-ΔG-MCh): the production of pseudotyped rabies virus was carried out as described previously [9] . Glycoprotein–gene-deleted rabies virus vector (Δgp-mCherry) was generated in which a mCherry (MCh) reporter gene was inserted into the locus encoding the rabies virus glycoprotein. The helper cell line, BHK-EnvARGCD, was infected with Δgp-mCherry, to produce rabies virus pseudotyped with envelope protein EnvA. After 2h and 4 h, the cells were washed with PBS three times and the media re-applied. Supernatants containing Δgp-mCherry rabies virus pseudotyped with EnvA were harvested 5 days later, filtered and concentrated by ultracentrifugation. Rabies virus titre was estimated to be ~1.2×10 E7 i.u. ml −1 and diluted for use to ~4×10E6 i.u. ml −1 . Stereotaxic surgery Mice were anaesthetised (Avertin 0.4 mg g −1 ) and stereotaxic surgery was performed to deliver 1 μl of retrovirus ( n =53) or lentivirus ( n =13) into the right DG using spatial coordinates relative to bregma as follows: AP=−2.10 mm; lateral=1.9 mm; ventral=2.10 mm, and AP=−3.10 mm; lateral=2.8 mm; ventral=3.10 mm. Rabies virus EnvA-ΔG-MCh (1 μl) was delivered in AP=−3.10 mm; lateral=2.8 mm; ventral=3.10 mm. These coordinates were modified from the mouse brain atlas [60] for mice aged 5–6 weeks at the time of injection. After 10–18 days, lentivirus-treated mice were injected with rabies virus EnvA-ΔG-MCh. The retrovirus-treated mice were injected with rabies virus EnvA-ΔG-MCh 7, 14, 21, 30, 60 or 90 days later. To test for non-specific labelling, rabies virus EnvA-ΔG-MCh only was injected into the DG ( n =3). The retrograde tracer Fluorogold (2% in 0.9% saline; Fluorochrome LLC) was infused in DG ( n =3) and mice perfused after 6 days. For lesion studies, mice were injected bilaterally into the PRH/LEC (coordinates: AP=−3.4 mm; lateral=4.3 mm; ventral=2.7 mm) or MEC (coordinates: AP=4.4 mm; lateral=3.2 mm; ventral=2.7 mm) with either 0.1 μl of NMDA (31.25 mM) dissolved in sterile PBS (0.1 M) or vehicle 1 week before electrophysiological recordings. For behavioural studies, PRH/LEC lesions (NMDA, n =10) or vehicle alone (PBS, n =16) were performed after the 'shaping' part of training in the touchscreen (see 'Behavioral testing' in the Supplementary Information ), and given 3 days to recover before task training and probe trials. For histological analysis, animals were given an overdose of anaesthetics and perfused trans-cardially with cold 4% paraformaldehyde (PFA) in 0.1 M PBS. After 24 h, brain tissue was equilibrated in 30% sucrose. Sequential sections (40 μm) were taken using a freezing microtome (HM450, ThermoFisher) through the entire brain and stored in phosphate-buffered glycerol at −20 °C. Immunocytochemistry and cell counts To identify the cell types innervating newborn neurons, labelling was carried out on 40-μm free-floating sections as described [27] . Primary antibodies, PV (mouse monoclonal; 1:1,000, Millipore), choline acetyltransferase (ChAT, goat polyclonal; 1:500, Millipore), calretinin (goat polyclonal, 1:500, Millipore), GFAP (rabbit polyclonal; 1:500, DAKO), GABA (rabbit polyclonal, 1:1,000, Sigma), somatostatin (rabbit polyclonal, 1:500, Peninsula Lab), neuropeptide Y (rabbit polyclonal, 1:500, Peninsula Lab), doublecortin (DCX; goat polyclonal, 1:500, Santa Cruz), BrdU (rat polyclonal, 1:100; Accurate Chemical), TVA (rabbit polyclonal, 1:100, kindly provided by Andrew Leavitt, UCSF); and Fluorogold (rabbit polyclonal, 1:1,000, Millipore) were applied. Corresponding fluorescent secondary antibodies (donkey anti-mouse CY5; donkey anti-goat CY5; donkey anti-rabbit CY5; donkey anti-rat CY3, Jackson ImmunoResearch) were used. Nuclei were visualized with 4′-6-diaminodino-2-phenylindole (DAPI). The number of hGFP + , double-labelled hGFP + -MCh + and MCh + -only cells, and double labelling of MCh + cells with markers for hilar cells was quantified in 1:12 series (480 μm apart) of horizontal sections (40 μm) through the dorsal–ventral extent of the brain. Imaging and microscopy Sections were evaluated (FV1000MPE, Olympus; SP5, Leica) and imaged with confocal microscopy (FV1000MPE, Olympus). In Supplementary Fig. S1 , spinning disc confocal microscope (CARV II, CrEST, Italy) images were stitched to produce a mosaic representing a single z plane (Metamorph, Molecular Devices). Ten or twelve z planes at 2-μm intervals were projected to generate representative panoramic images. For high-magnification images X60 and X×100 objectives (PlanApoN, ×60, 1.42, and PlanSApo, ×100, 1.40; Olympus) were used at 0.5–1 μm intervals. Z-series were merged and processed using Slidebook (Intelligent Imaging Innovations) and Photoshop (Adobe). Excitotoxic lesions were evaluated using light microscopy (BX51, Olympus) and StereoInvestigator (Microbrightfield) was used to trace the outline of, and reconstruct (CorelDraw), the PRH/LEC lesioned areas. Electrophysiology Mice ( n =53) were anaesthetised with isoflurane and decapitated. Brains were removed into a chilled solution containing (in mM): 110 Choline-Cl − , 2.5 KCl, 2 NaH 2 PO 4 , 25 NaHCO 3 , 20 glucose, 0.5 CaCl 2 , 7 MgCl 2 , 0.6 Na + pyruvate, 1.3 Na + ascorbate, 1 kynurenic acid. Horizontal entorhinal cortex-hippocampus slices (400 μm thick) were obtained and transferred to a chamber containing artificial cerebrospinal fluid (ACSF) in mM: 125 NaCl, 2.5 KCl, 2 NaH 2 PO 4 , 25 NaHCO 3 , 2 CaCl 2 , 1.3 MgCl 2 , 10 glucose, 3.1 Na + pyruvate, 1.3 Na + ascorbate, bubbled with 95% O 2 /5% CO 2 (pH 7.4, 310 mOsm), and stored at 30 °C during recovery. Recordings were carried out in ACSF at 28±1 °C using microelectrodes (3–5 MΩ) pulled from borosilicate glass (G150F-4, Warner Instruments) and filled with (in mM): 120 K-gluconate, 20 KCl, 5 NaCl, 4 MgCl 2 , 0.1 EGTA, 10 HEPES, 4 Tris-ATP, 10 phosphocreatine (pH 7.4, 295 mOsm). GFP + and MCh + cells were identified under epifluorescence and visualized with infra-red differential interference contrast video microscopy (Olympus BX51WI). Mature GCs were recorded from the outer portion of the granule cell layer. Whole-cell patch-clamp recordings (Multiclamp 700B, Axon Instruments) were filtered at 2 kHz and digitalized at 20 kHz (Digidata 1322A and pClamp 10.2 Software; Molecular Devices). Recordings were not corrected for a liquid junction potential. Series resistance was typically 10–30 MΩ. Resting potentials were measured immediately after break-in. Extracellular stimulation (10 μs, 0.05 Hz; Grass S88 stimulator and isolation unit, Grass Instrument) was done using pipettes (2–4 MΩ) filled with ACSF placed in the middle third and outer molecular layer at >250 μm from the recorded cell. The holding potential was set at −80 mV. Bicuculline methiodide (20 μM, Sigma) was added in plasticity (paired-pulse) experiments. Data analysis: the R in was measured using a linear regression of voltage deflections (±15 mV resting potential, ~−75 mV) in response to 600 ms current steps of 6–10 different amplitudes (increments, 5 pA). The τ m was calculated fitting a single exponential function from the mean responses to 20 successive hyperpolarizing current pulses (−10 pA; 500 ms). C m was calculated according to C m = τ m / R m . AP amplitude was defined as the difference in membrane potential between threshold and the peak. After-hyperpolarization (AHP) amplitude was defined as the difference between AP threshold and the most-negative membrane potential attained during the AHP. Firing frequency was calculated as the inverse of the mean inter-spike interval of the first two inter-spike intervals of the train. Peak of the EPSCs was measured from the holding potential. Rise time was calculated from 10–90% of the peak amplitude. How to cite this article: Vivar, C. et al . Monosynaptic inputs to new neurons in the dentate gyrus. Nat. Commun. 3:1107 doi: 10.1038/ncomms2101 (2012).